ACS-20/FATP4 mediates the anti-ageing effect of dietary restriction inC. elegans 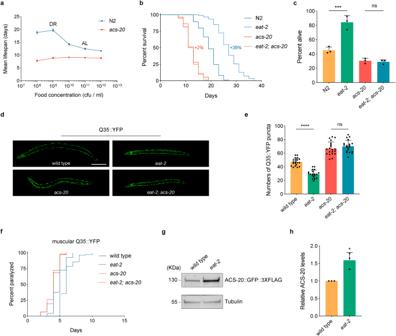Fig. 1: ACS-20 is required for DR-induced lifespan and healthspan extension. aMean lifespan of the wild-type N2 andacs-20mutant fed with bacterial food at different concentrations (1.0 × 108–1.0 × 1012cfu/ml). Data are represented as mean ± SD based on three independent experiments. AL,ad libitum(1.0 × 1011cfu/ml), DR, optimal dietary restriction condition (1.0 × 109cfu/ml).bSurvival curves of N2,eat-2,acs-20, andeat-2; acs-20mutant animals. Percentages indicate changes in mean lifespan induced by theeat-2mutation. N2 vs.eat-2,p< 0.0001;acs-20vs.eat-2; acs-20,p= 0.8271 (log-rank tests).cSurvival percentages of N2,eat-2,acs-20, andeat-2; acs-20mutant animals incubated at 35 °C for 10 h. Data are represented as mean ± SD (n= 3). ***p< 0.001; ns,p= 0.9875 (One-way ANOVA with Turkey’s multiple comparisons test).d,eRepresentative photographs of 3-day-old adult wild-type,eat-2,acs-20andeat-2; acs-20mutant animals expressing the muscular Q35::YFP (d) and quantification of the Q35::YFP punctae (e). Data are represented as mean ± SD (n= 20). ****p< 0.0001; ns,p= 0.5231 (One-way ANOVA with Turkey’s multiple comparisons test). Scale bar, 100 μm.fParalysis of wild-type,eat-2,acs-20andeat-2; acs-20mutant animals expressing the muscular Q35::YFP. Wild-type vs.eat-2,p< 0.0001;acs-20vs.eat-2; acs-20,p= 0.2364 (log-rank tests).g,hImmunoblots (g) and quantification (h) of ACS-20::GFP::3✕FLAG and tubulin protein levels in the wild type andeat-2mutant. The ratio of band intensity of ACS-20::GFP::3✕FLAG to tubulin was normalized to the wild type. Data are represented as mean ± SD (n= 3). *p= 0.0111 (two-tailedt-test). Source data are provided as a Source Data file. Dietary restriction is an effective anti-ageing intervention across species. However, the molecular mechanisms from the metabolic aspects of view are still underexplored. Here we show ACS-20 as a key mediator of dietary restriction on healthy ageing from a genetic screen of the C. elegans acyl-CoA synthetase family. ACS-20 functions in the epidermis during development to regulate dietary restriction-induced longevity. Functional transcriptomics studies reveal that elevated expression of PTR-8/Patched is responsible for the proteostasis and lifespan defects of acs-20 . Furthermore, the conserved NHR-23 nuclear receptor serves as a transcriptional repressor of ptr-8 and a key regulator of dietary restriction-induced longevity. Mechanistically, a specific region in the ptr-8 promoter plays a key role in mediating the transcription regulation and lifespan extension under dietary restriction. Altogether, these findings identify a highly conserved lipid metabolism enzyme as a key mediator of dietary restriction-induced lifespan and healthspan extension and reveal the downstream transcriptional regulation mechanisms. Numerous studies have demonstrated that ageing can be modulated by highly conserved genes and pathways, and the molecular mechanisms involve the interaction with environmental factors such as nutrients [1] . Besides the genetic modulation of ageing, environmental changes can also have a significant impact on ageing. Dietary restriction (DR), reduced food intake without malnutrition, is one of the most robust environmental interventions that not only extend lifespan but also improve healthspan [2] , [3] , [4] . Originally reported in a study that rats with reduced food intake had significantly increased longevity [5] , DR has been shown to prolong the longevity of S. cerevisiae [6] , [7] , C. elegans [8] , Drosophila [9] , as well as M. mulatta [10] . Although there has not been direct evidence to connect DR with human longevity, many studies showed the beneficial effects of DR in human health [4] . Thus, it is of high significance to investigate the molecular mechanisms of DR in model animals for common downstream targets, which can be subject to pharmaceutical interventions to delay ageing. Genetic studies using model animals have helped to reveal the molecular mechanisms of DR. Several DR methods have been developed using C. elegans as a model [2] , [3] . Hypomorphic mutants of eat-2 , which encodes a subunit of the nicotinic acetylcholine receptor, have reduced food in-take thus serving as a genetic mimic of DR [8] . DR can be achieved by directly manipulating the bacterial food, such as feeding animals with diluted food either in liquid culture [11] , [12] or on solid agar plates [13] , [14] , complete food deprivation [15] , and intermittent fasting [16] . Using these DR regimens, researchers have identified multiple mediators of DR-induced longevity, including transcription factors SKN-1/Nrf2 [12] , PHA-4/FOXA [11] , DAF-16/FOXO [13] , HSF-1/HSF [15] , and NHR-62/HNF4α [17] , stress regulators EGL-9/PHD [14] and IRE-1/IRE [14] , energy homeostasis regulator AAK-2/AMPKα [13] and so on. Mutations in these regulators either completely or largely block DR-induced longevity. The downstream mechanisms of DR involve mitochondrial functions, various stress responses, autophagy, proteostasis, and metabolism [11] , [12] , [13] , [15] , [16] , [18] , [19] . Although lipid metabolism plays important roles in ageing and health, it has not been clear whether specific enzymes from the complex lipid metabolic network are required for the anti-ageing effect of DR. The acyl-CoA synthases (ACSs) family of enzymes function in the initial step of fatty acid metabolism by catalyzing the synthesis of fatty acyl-CoAs, which serve as metabolic intermediates [20] to enter subsequent lipid metabolic processes, such as lipid synthesis and degradation, lipid modification of proteins, and generation of transcriptional regulators and signaling molecules. In C. elegans , there are 21 acs genes ( acs −1–7, 9-22), many of which have not been well characterized for their roles in lipid metabolism or other biological processes. In this study, we set out to examine whether the acs genes are required for the DR-induced lifespan extension by an RNAi-based genetic screen. We found that ACS-20 is required for the lifespan and healthspan extension by DR. Spatiotemporal analysis reveals that ACS-20 functions in the epidermis during development to regulate DR-induced longevity. Functional genomics studies demonstrate that the acs-20 mutation leads to ER stress under DR. ptr-8 , which encodes an ortholog of Patched from the Hedgehog pathway, is transcriptionally upregulated in the acs-20 mutant, and it is responsible for the lifespan and proteostasis defects of the acs-20 mutant under DR. Studies on the transcriptional regulation show that the NHR-23/RORA nuclear hormone receptor serves as not only a transcriptional repressor of ptr-8 , but also a key mediator of DR-induced longevity. Moreover, a specific region of the ptr-8 promoter has been mapped as an important cis -regulatory element for the NHR-23-mediated transcriptional regulation of ptr-8 . Deletion of this region alleviates the DR-induced longevity defect when animals are subject to acs-20 or nhr-23 knockdown. Therefore, ACS-20 functions through NHR-23 to restrict the expression of PTR-8 to ensure the beneficial effects of DR on lifespan and healthspan. ACS-20 is a key mediator of DR-induced lifespan and healthspan extension To characterize the roles of lipid metabolism in the anti-ageing effect of DR, we performed an RNAi-based genetic screen of 21 acyl-CoA synthetase ( acs ) genes for their effects on lifespan under DR conditions in C. elegans . Compared to the control RNAi, the acs-20 RNAi treatment most significantly suppresses the prolonged longevity by DR (Supplementary Fig. 1 ). acs-20 encodes the C. elegans ortholog of the fatty acid transporter 4 (FATP4), mutations in which leads to abnormal lipid metabolism in the epidermis and disease such as ichthyosis prematurity syndrome (IPS) in mammals [21] , [22] . In C. elegans , the acs-20 mutant shows abnormalities in cuticle structures [23] . To further validate the role of ACS-20 in DR-induced lifespan extension, wild-type N2 and acs-20 deletion mutant animals were treated with bacterial food at different concentrations (1.0 × 10 8 –1.0 × 10 12 cfu/ml) from day 1 adulthood for survival assays. Unlike N2 animals, which exhibit more lifespan extension with food dilution until the optimal DR condition (1.0 × 10 9 cfu/ml), the acs-20 mutant shows no significant changes in lifespan under different nutrient conditions (Fig. 1a ). The eat-2 mutant, which has reduced feeding and significantly extended lifespan, has been widely used as a genetic mimic of DR [8] . The acs-20 mutant completely abolishes the prolonged longevity of eat-2 animals (Fig. 1b ). Therefore, ACS-20 is a key mediator of DR-induced longevity. Fig. 1: ACS-20 is required for DR-induced lifespan and healthspan extension. a Mean lifespan of the wild-type N2 and acs-20 mutant fed with bacterial food at different concentrations (1.0 × 10 8 –1.0 × 10 12 cfu/ml). Data are represented as mean ± SD based on three independent experiments. AL, ad libitum (1.0 × 10 11 cfu/ml), DR, optimal dietary restriction condition (1.0 × 10 9 cfu/ml). b Survival curves of N2, eat-2 , acs-20 , and eat-2; acs-20 mutant animals. Percentages indicate changes in mean lifespan induced by the eat-2 mutation. N2 vs. eat-2 , p < 0.0001; acs-20 vs. eat-2; acs-20 , p = 0.8271 (log-rank tests). c Survival percentages of N2, eat-2 , acs-20 , and eat-2; acs-20 mutant animals incubated at 35 °C for 10 h. Data are represented as mean ± SD ( n = 3). *** p < 0.001; ns, p = 0.9875 (One-way ANOVA with Turkey’s multiple comparisons test). d , e Representative photographs of 3-day-old adult wild-type, eat-2 , acs-20 and eat-2; acs-20 mutant animals expressing the muscular Q35::YFP ( d ) and quantification of the Q35::YFP punctae ( e ). Data are represent e d as mean ± SD ( n = 20). **** p < 0.0001; ns, p = 0.5231 (One-way ANOVA with Turkey’s multiple comparisons test). Scale bar, 100 μm. f Paralysis of wild-type, eat-2 , acs-20 and eat-2; acs-20 mutant animals expressing the muscular Q35::YFP. Wild-type vs. eat-2 , p < 0.0001; acs-20 vs. eat-2; acs-20 , p = 0.2364 (log-rank tests). g , h Immunoblots ( g ) and quantification ( h ) of ACS-20::GFP::3✕FLAG and tubulin protein levels in the wild type and eat-2 mutant. The ratio of band intensity of ACS-20::GFP::3✕FLAG to tubulin was normalized to the wild type. Data are represented as mean ± SD ( n = 3). * p = 0.0111 (two-tailed t -test). Source data are provided as a Source Data file. Full size image In addition to lifespan, healthspan is also an important assessment of healthy ageing [1] . To explore the role of acs-20 in healthspan regulation, we first examined thermotolerance phenotypes of N2, eat-2 , acs-20 , and eat-2; acs-20 mutants by heat shock at 35 °C for 10 h. The eat-2 mutant shows significantly increased resistance to the heat stress compared to the wild-type N2, whereas the acs-20 mutation completely blocks the protective effect of eat-2 (Fig. 1c ). Polyglutamine (polyQ) expansion-induced proteotoxicity has been linked with several degenerative diseases [24] . We took advantage of an established polyQ model, in which a transgene expresses polyQ (Q35) fused with YFP in the body wall muscle [25] , to test the effect of acs-20 on proteostasis. Compared to the wild type, the eat-2 mutant shows significantly less Q35::YFP aggregates and delayed paralysis due to the proteotoxicity in body wall muscle cells (Fig. 1d–f ). However, the protective effect of eat-2 is abrogated by the acs-20 mutation (Fig. 1d–f ). Taken together, these results demonstrate that ACS-20 is required for DR-induced healthspan extension. To further examine whether ACS-20 is regulated by nutrients, we performed CRISPR/Cas9-based genome editing experiment to knock in GFP::3 ✕ FLAG coding sequence to the 3′ end of acs-20 . We then compared ACS-20 protein levels between wild-type and eat-2 mutant animals via immunoblots. The ACS-20::GFP::3 ✕ FLAG protein levels are mildly but significantly elevated under DR (Fig. 1g, h ), suggesting ACS-20 is involved in the response to low nutrient conditions. Temporospatial requirement of ACS-20 in DR-induced longevity The acs-20::gfp::3 x flag knockin (KI) strain allows us to characterize the endogenous expression patterns of ACS-20. Confocal microscopy images show that ACS-20 is mainly expressed in the epidermal and muscular tissues (Fig. 2a ), with the expression levels significantly diminished during adulthood (Fig. 2b ). RT-qPCR measurement of the endogenous acs-20 mRNA levels confirms that acs-20 expression levels in adulthood are significantly lower than those in the third (L3) or fourth (L4) larval stages (Fig. 2c ). Thus, acs-20 is expressed in a temporospatial manner. Fig. 2: ACS-20 functions in the epidermis during development to regulate DR-induced lifespan extension. a Representative photographs of the endogenous ACS-20::GFP::3✕FLAG expression in different tissues. Scale bar, 20 μm. b Representative photographs of ACS-20::GFP expression in the fourth larval stage (L4) and day 1 adulthood. Scale bar, 50 μm. c RT-qPCR quantification of acs-20 mRNAs at different stages. Data are represented as mean ± SD ( n = 3). ns, p = 0.9880; *** p < 0.001 (One-way ANOVA with Turkey’s multiple comparisons test). d , e Survival curves of N2 and eat-2 mutant animals treated with the global control or acs-20 RNAi in whole life ( d ) or adulthood ( e ). N2 vs. e at-2 with the control RNAi treatment, p < 0.0001 (whole life, adulthood); N2 vs. eat-2 with the acs-20 RNAi treatment, p = 0.3093 (whole life), p < 0.0001 (adulthood) (log-rank tests). f , g Survival curves of wild type (wt) and eat-2 mutant animals treated with the epidermal ( f ) or muscular ( g ) control or acs-20 RNAi. wt vs. eat-2 with the control RNAi treatment, p < 0.0001 (epidermal RNAi, muscular RNAi); wt vs. eat-2 with the acs-20 RNAi treatment, p = 0.0662 (epidermal RNAi), p < 0.0001 (muscular RNAi) (log-rank tests). h Survival curves of acs-20 and eat-2; acs-20 mutants with or without the acs-20 transgene driven by the epidermis-specific dpy-7 promoter. acs-20 vs. eat-2; acs-20 , p = 0.9773 (without the transgene), p < 0.0001 (with the transgene) (log-rank tests). Percentages indicate changes in mean lifespan induced by the eat-2 mutation. Source data are provided as a Source Data file. Full size image To determine when and where ACS-20 functions to regulate lifespan under DR, we performed RNAi knockdown experiments to examine the effects of acs-20 reduced function on longevity. Consistent with the temporal expression patterns, the whole life acs-20 RNAi treatment completely abolishes DR-induced lifespan extension (Fig. 2d ), whereas acs-20 RNAi only during adulthood has little effect on lifespan (Fig. 2e ). Suppression of DR-induced longevity can also be achieved by the epidermis-specific acs-20 RNAi treatment (Fig. 2f ), but not by muscle-specific acs-20 RNAi (Fig. 2g ). To validate these findings, a single-copy transgene of acs-20 driven by its own promoter was constructed for rescue experiments. The DR-induced lifespan extension deficiency of acs-20 is fully restored by this transgene (Supplementary Fig. 2 ). Another single-copy transgene of acs-20 driven by the dpy-7 promoter, which is specifically active in the epidermis only during development [26] , also completely restored DR-induced longevity in the acs-20 mutant background (Fig. 2h ). Collectively, ACS-20 functions in the epidermis during developmental stages to regulate DR-induced longevity. Effects of acs-20 on lipid metabolism ACS-20 is orthologous to the mammalian FATP4, which serves predominantly as an acyl-CoA synthetase rather than a fatty acid transporter [27] . Mutations in humans or mice FATP4 lead to lipid metabolic defects in the skin [21] , [22] . To characterize whether the acs-20 mutant affects lipid accumulation, we performed Oil Red O (ORO) staining to measure neutral lipid levels in the intestine, the major metabolic and lipid storage tissue in C. elegans . Imaging and quantification results demonstrate that the acs-20 mutation does not affect the intestinal lipid levels compared to the wild-type N2, whereas the eat-2; acs-20 mutant has slightly increased lipid accumulation compared to the eat-2 mutant (Supplementary Fig. 3a, b ). Since ACS-20 functions in the epidermis, another lipid storage tissue in C. elegans , to regulate lifespan, it is important to examine whether the acs-20 mutation affects lipid accumulation in the epidermis. However, the ORO staining method with fixed animals does not allow quantitative assessment of epidermal lipid droplets. Previous studies have shown that DGAT-2 is a membrane protein of lipid droplets, and a single-copy gfp::dgat-2 transgene driven by the intestine-specific vha-6 promoter can be used for quantitative measurement of intestinal lipid droplets [28] . We then constructed a single-copy gfp::dgat-2 transgene driven by the epidermis-specific col-12 promoter. Imaging and quantification assays show that the acs-20 mutation does not affect epidermal lipid droplet levels either in the wild type or in the eat-2 mutant background (Supplementary Fig. 3c, d ). Altogether, these results suggest that ACS-20 might not regulate DR-induced lifespan extension via affecting lipid accumulation in metabolic tissues. Functional transcriptomics analysis of the acs-20 mutant To gain mechanistic insights of ACS-20 for its role in ageing, we conducted transcriptional profiling of the wild-type N2, acs-20, eat-2 , and eat-2; acs-20 mutant animals via mRNA-Seq. Bioinformatic analysis reveals that with the cutoff at fold changes >2 and adjusted p < 0.01, there are 61 upregulated and 45 down-regulated genes in acs-20 compared to N2, whereas there are 138 upregulated and 38 down-regulated genes in eat-2; acs-20 compared to eat-2 (Fig. 3a and Supplementary Data 1 ). The 95 genes that are significantly upregulated in eat-2; acs-20 compared to eat-2 but show no significant changes in acs-20 compared to N2 were used for Gene Ontology (GO) analysis as these genes are more likely to be involved in the DR-specific response (Fig. 3b ). The most significantly enriched GO term is endoplasmic reticulum (ER) unfolded protein response (Fig. 3c ). Fig. 3: The acs-20 mutation causes ER stress under DR. a Volcano plots of differentially expressed genes in the acs-20 vs. N2 and eat-2; acs-20 vs. eat-2 data sets. Red and blue points represent genes with significantly increased or decreased expression, respectively ( p < 0.01, Wald tests with Bonferroni corrections). b A Venn diagram comparing genes upregulated in eat-2; acs-20 vs. eat-2 and genes not differentially expressed in acs-20 vs. N2. c Significantly enriched Gene Ontology (GO) terms (hypergeometric tests with Benjamini-Hochberg corrections) for genes significantly upregulated in the eat-2; acs-20 mutant compared to the eat-2 mutant. d RT-qPCR quantification of abu genes in eat-2 and eat-2; acs-20 mutant animals. Data are represented as mean ± SD ( n = 3). **** p < 0.0001; *** p < 0.001; ** p < 0.01; * p < 0.05; ns, p = 0.0598 (two-tailed t -tests). e , f Representative photographs of the ER stress reporter hsp-4p::gfp expression in wild-type, acs-20 , eat-2 , and eat-2; acs-20 animals treated with DMSO or tunicamycin ( e ) and quantification of the GFP fluorescence intensities (a.u. arbitrary unites). Data are represented as mean ± SD ( n = 10). **** p < 0.0001; ns, acs-20 p > 0.9999, eat-2; acs-20 p = 0.9993 (One-way ANOVA with Turkey’s multiple comparisons test). Scale bar, 200 μm. g Percentages of N2, acs-20 , eat-2 , and eat-2; acs-20 mutant animals that died (dead), developmentally arrested (L1-L3) or completed development (L4) upon 0, 0.25 or 0.50 μg/ml tunicamycin treatments. Data are represented as mean ± SD ( n = 3). For animals that completed development upon tunicamycin treatment, N2 vs. acs-20 , p < 0.01; eat-2 vs. eat-2; acs-20 , p < 0.0001 (Two-way ANOVA with Turkey’s multiple comparisons test). Source data are provided as a Source Data file. Full size image RT-qPCR experiments confirmed the mRNA-Seq results that mRNA levels of multiple ER stress-related abu genes are significantly elevated in the eat-2; acs-20 double mutant compared to the eat-2 mutant (Fig. 3d ). abu genes encode endomembrane proteins, the expression of which is induced in ER-stressed animals when the IRE-1–XBP-1 ER unfolded protein response (ER UPR ) pathway is inactivated [29] . Tunicamycin is a protein N-glycosylation inhibitor which induces ER stress [30] . The tunicamycin treatment leads to robust activation of the hsp-4::gfp reporter, which has been widely used to monitor the ER UPR activation in C. elegans . Intriguingly, tunicamycin cannot activate hsp-4::gfp expression when acs-20 is mutated either under normal feeding or DR conditions (Fig. 3e, f ), suggesting the acs-20 mutant might have reduced capability to deal with ER stress. Consistently, tunicamycin treatments cause more severe developmental delay and lethality when acs-20 is deleted in the wild-type or eat-2 mutant background (Fig. 3g ). Dithiothreitol (DTT) and thapsigargin are also ER stressors that function via affecting the ER lumen oxidative environment [31] and causing ER Ca 2+ depletion [32] , respectively. DTT or thapsigargin treatment leads to more severe developmental defects in the acs-20 and eat-2; acs-20 mutants compared to the wild-type N2 and eat-2 mutant, respectively (Supplementary Fig. 4 ). These results suggest that the acs-20 mutation might compromise proteostasis thus increasing the sensitivity to ER stress, which contributes to the lifespan and healthspan defects under DR. PTR-8/Patched as a key mediator of acs-20 for its roles in longevity and proteostasis regulation under DR It is plausible that genes upregulated in the eat-2; acs-20 double mutant are responsible for the lifespan and proteostasis defects of acs-20 under DR. Therefore, we performed an RNAi screen in the eat-2; acs-20 double mutant background to individually knock down the 95 genes that are specifically upregulated by the acs-20 mutant under DR for lifespan extension phenotypes. Knockdown of ptr-8 , which encodes an ortholog of the Hedgehog receptor, significantly extends lifespan of the eat-2; acs-20 mutant. We then constructed a ptr-8 knockout (KO) mutant via CRISPR/Cas9. In the acs-20 mutant, DR induces significant lifespan extension in the absence of PTR-8 ( ptr-8; acs-20 vs. ptr-8 eat-2; acs-20 ) compared to the controls ( acs-20 vs. eat-2; acs-20 ), which show no significant DR-mediated changes in lifespan (Fig. 4a ). In addition, RT-qPCR assays confirmed that compared to the eat-2 mutant, the ptr-8 mRNA levels are robustly elevated by nearly 10-fold in the eat-2; acs-20 double mutant, whereas the difference between N2 and acs-20 mutant is not significant (Fig. 4b ). Furthermore, the ptr-8 deletion reduces mRNA levels of ER stress-related abu genes in eat-2; acs-20 compared to eat-2 (Fig. 4c ), and significantly increases the resistance to various ER stressors including tunicamycin, DTT, and thapsigargin in the eat-2; acs-20 mutant (Fig. 4d and Supplementary Fig. 4 ). Fig. 4: Elevated PTR-8 expression in acs-20 disrupts the protective effect of DR on lifespan and proteostasis. a Survival curves of acs-20 , eat-2; acs-20 , ptr-8; acs-20 , and ptr-8 eat-2; acs-20 . acs-20 vs. eat-2; acs-20 , p = 0.0995; ptr-8; acs-20 vs. ptr-8 eat-2; acs-20 , p < 0.0001 (log-rank tests). Percentages indicate changes in mean lifespan induced by eat-2 . b RT-qPCR quantification of ptr-8 mRNAs in N2, acs-20 , eat-2 , and eat-2 ; acs-20 . Data are represented as mean ± SD ( n = 3). **** p < 0.0001; ns, p = 0.7886 (One-way ANOVA with Turkey’s multiple comparisons test). c RT-qPCR quantification of abu genes in eat-2; acs-20 and ptr-8 eat-2; acs-20 . Data are represented as mean ± SD ( n = 3). **** p < 0.0001; *** p < 0.001; ** p < 0.01 (two-tailed t -tests). d Percentages of N2, acs-20 , eat-2 , eat-2; acs-20 , ptr-8 , ptr-8; acs-20 , ptr-8 eat-2 , and ptr-8 eat-2; acs-20 that died (dead), developmentally arrested (L1-L3) or completed development (L4) upon 0, 0.25 or 0.50 μg/ml tunicamycin treatment. Data are represented as mean ± SD ( n = 3). For animals that completed development upon tunicamycin treatment, eat-2 vs. eat-2; acs-20 , p < 0.0001; eat-2; acs-20 vs. ptr-8 eat-2; acs-20 , p < 0.0001 (Two-way ANOVA with Turkey’s multiple comparisons test). e , f Representative photographs of wild-type, acs-20 , eat-2 , and eat-2; acs-20 animals expressing muscular Q35::YFP treated with the control or ptr-8 RNAi ( e ) and quantification of the Q35::YFP punctae ( f ). Data are represented as mean ± SD ( n = 10). **** p < 0.0001; ** p < 0.01 (One-way ANOVA with Turkey’s multiple comparisons test). Scale bar, 100 μm. g Paralysis analysis of the wild-type, eat-2 , acs-20 , and eat-2; acs-20 mutant animals expressing muscular Q35::YFP with control or ptr-8 RNAi. **** p < 0.0001; ns, p > 0.05 (log-rank tests). h , i Immuno-blots ( h ) and quantification ( i ) of the SDS-resistant Q35::YFP aggregates, total Q35::YFP, and tubulin in the wild-type, eat-2 , acs-20 , and eat-2; acs-20 with control or ptr-8 RNAi. Data are represented as mean ± SD ( n = 3). ** p < 0.01; ns, p > 0.05 (One-way ANOVA with Turkey’s multiple comparison tests). Source data are provided as a Source Data file. Full size image Since the ptr-8 deletion significantly abrogates the ER stress response in eat-2; acs-20 , we then set out to characterize the role of PTR-8 in proteostasis using the transgenic polyQ model. Imaging and quantification experiments show that compared to the control RNAi, the ptr-8 RNAi treatment significantly reduces the amount of the Q35::YFP aggregates in the eat-2; acs-20 double mutant (Fig. 4e, f ). Consistently, the ptr-8 RNAi treatment also significantly delays age-related paralysis caused by the Q35::YFP aggregation (Fig. 4g ). To make more quantitative assessment of DR, acs-20 , and ptr-8 for their roles in proteostasis, we performed filter trap assays and immunoblots to measure aggregated and total Q35::YFP respectively in the wild-type, eat-2 , acs-20 , and eat-2; acs-20 animals treated with the control or ptr-8 RNAi (Fig. 4h ). Quantification analysis shows that compared to the wild-type animals, the DR-mimicking eat-2 mutant has significantly less Q35::YFP aggregation, whereas this effect is abolished by the acs-20 mutation (Fig. 4i ). On the other hand, inhibition of ptr-8 restores the protective effect of DR as indicated by significantly reduced levels of Q35::YFP aggregates in the eat-2; acs-20 mutant treated with the ptr-8 RNAi compared to the control RNAi (Fig. 4h, i ). Altogether, these results demonstrate that PTR-8 functions downstream of acs-20 as a key regulator of proteostasis and longevity under DR. NHR-23/RORA functions downstream of acs-20 to repress ptr-8 transcription Since the ptr-8 mRNA levels are significantly elevated in the eat-2; acs-20 mutant, we constructed a reporter strain that carries a 3 kb ptr-8 promoter driving gfp transgene to study the transcriptional regulation mechanisms. This reporter strain shows GFP expression mainly in the epidermis, and the epidermal GFP signal is significantly increased in the eat-2; acs-20 mutant compared to the wild type (Fig. 5a ). These expression patterns suggest that there might be either transcriptional repressors that restrict ptr-8 expression in the wild-type background, or transcriptional activators that promote ptr-8 expression in the eat-2; acs-20 mutant. To test these hypotheses, we performed genetic screens for altered ptr-8p::gfp expression using the transcription factor RNAi sub-library in the wild-type and eat-2; acs-20 mutant backgrounds, respectively. Although we did not find any RNAi treatment that reduces the high level of ptr-8p::gfp expression in eat-2; acs-20 , we identified NHR-23 as a transcriptional repressor of ptr-8 in the wild type as RNAi knockdown of nhr-23 increases not only expression levels of the ptr-8p::gfp reporter (Fig. 5b ), but also endogenous ptr-8 mRNA levels as quantified via RT-qPCR (Fig. 5c ). nhr-23 encodes a nuclear hormone receptor that is orthologous to RORA, a key transcriptional regulator of the circadian clock [33] . Like acs-20 , epidermis-specific RNAi knockdown of nhr-23 also significantly blocks DR-induced lifespan extension (Fig. 5d ). Fig. 5: NHR-23/RORA mediates the effect of acs-20 on ptr-8 expression and lifespan. a Representative photographs of the ptr-8 p(3k)::GFP reporter expression in wild-type and eat-2; acs-20 animals. Scale bar, 50 μm. b Representative photographs of the ptr-8 p(3k)::GFP expression in animals treated with the control or nhr-23 RNAi. Scale bar, 200 μm. c RT-qPCR quantification of ptr-8 mRNA levels in wild-type animals treated with the control or nhr-23 RNAi. Data are represented as mean ± SD ( n = 3). ** p = 0.0084 (two-tailed t -test). d Survival curves of wild type (wt) and eat-2 mutant animals treated with the epidermis-specific control or nhr-23 RNAi. wt vs. eat-2 : control RNAi, p < 0.0001; nhr-23 RNAi, p < 0.01 (log-rank tests). e Representative photographs of the ptr-8 p(Δ1.5-3 k)::GFP, ptr-8 p(Δ2.7-3 k)::GFP, ptr-8 p(Δ1.9-2.7 k)::GFP, and ptr-8 p(Δ1.5-1.8 k)::GFP expression in animals treated with the control or nhr-23 RNAi. Scale bar, 200 μm. f , g RT-qPCR quantification of ptr-8 mRNA levels in N2 and the ptr-8 p(Δ1.9-2.7 k) mutant animals treated with either control vs. nhr-23 RNAi ( g ) or control vs. acs-20 RNAi ( h ). Data are represented as mean ± SD ( n = 3). **** p < 0.0001; ns, p = 0.9972 ( nhr-23 RNAi), p = 0.9972 ( acs-20 RNAi) (One-way ANOVA with Turkey’s multiple comparisons test). h ChIP-qPCR quantification of the relative enrichment of NHR-23::GFP binding with the ptr-8 promoter region (1861–1958 bp) in N2, acs-20 , eat-2 and eat-2; acs-20 . The fold enrichment was normalized by the input DNA. Data are represented as mean ± SD ( n = 3). ****, p < 0.0001 (two-tailed t -tests). i , j Survival curves of ptr-8 p(Δ1.9-2.7 k) and ptr-8 p(Δ1.9-2.7 k) eat-2 mutant animals treated with the control vs. nhr-23 RNAi ( i ) or acs-20 RNAi ( j ). ptr-8 p(Δ1.9–2.7 k) vs. ptr-8 p(Δ1.9–2.7 k) eat-2 : control RNAi, p < 0.0001; nhr-23 RNAi, p < 0.0001; acs-20 RNAi, p < 0.0001 (log-rank tests). Percentages indicate changes in mean lifespan induced by the eat-2 mutant. Source data are provided as a Source Data file. Full size image To further characterize the transcriptional regulation of ptr-8 by NHR-23, we constructed transgenic lines carrying serial deletions of ptr-8 promoter:: gfp reporters. In contrary to the 3 kb promoter, the ptr-8 p(Δ1.5-3k):: gfp reporter does not respond to nhr-23 RNAi knockdown (Fig. 5e ), suggesting the key cis -regulatory element is located within the 1.5–3 kb region of the ptr-8 promoter. Further studies narrow the cis -regulatory element down to the 1.9–2.7 kb region of the ptr-8 promoter (Fig. 5e ). We then set out to investigate whether the identified promoter region is functional regarding to the regulation of ptr-8 transcription and longevity in vivo. CRISPR/Cas9-based genome editing was performed to create a 833-bp deletion mutant of the 1.9–2.7 kb ptr-8 promoter region. RT-qPCR experiments reveal that the significantly elevated ptr-8 expression upon nhr-23 or acs-20 RNAi treatment is completely blocked in the absence of this promoter region (Fig. 5f, g ). To examine whether NHR-23 interacts with the ptr-8 promoter region, we performed genome editing experiment to create the nhr-23::gfp knockin strain. ChIP-qPCR using anti-GFP antibodies show that NHR-23::GFP has reduced interaction with the ptr-8 promoter in the absence of ACS-20 (Fig. 5h ). Moreover, deletion of the 1.9–2.7 kb ptr-8 promoter region is sufficient to restore DR-induced lifespan extension when animals are subjected to nhr-23 or acs-20 RNAi knockdown (Fig. 5i, j ). NHR-23 does not seem to be the only ACS-20 downstream transcriptional regulator of ptr-8 since deletion of the 1.9–2.7 kb ptr-8 promoter region is not sufficient to increase ptr-8 expression (Fig. 5e–g ) or block DR-induced lifespan expression (Fig. 5i, j ). One plausible model is that NHR-23 functions through inhibiting a transcriptional activator of ptr-8 rather than directly represses ptr-8 expression (Fig. 6 ). When the cis -regulatory element is deleted, neither NHR-23 or the unknown factor can affect ptr-8 expression. Animals thus show normal response to DR. Taken together, these results demonstrate that NHR-23 functions downstream of ACS-20 to repress ptr-8 expression and ensure DR-induced lifespan extension. Fig. 6: Schematic representation on the regulation of DR-induced healthy ageing by ACS-20, NHR-23, and PTR-8. ACS-20 functions in the epidermis during development to regulate DR-induced lifespan extension. In the presence of ACS-20, the NHR-23/RORA nuclear hormone receptor functions with an unknown factor to restrict the expression of PTR-8/Patched via a cis -regulatory element to maintain proteostasis and promote healthy ageing under DR. In the absence of ACS-20, NHR-23-mediated transcriptional repression of ptr-8 is abolished. Overexpression of PTR-8 results in disrupted proteostasis and elevated ER stress, which block the lifespan extension produced by DR. Full size image In summary, we have identified ACS-20/FATP4 as a key mediator of DR on healthy ageing from a targeted genetic screen. ACS-20 functions in the epidermis during development to regulate DR-induced lifespan extension. Under DR, ACS-20 functions through the NHR-23/RORA nuclear hormone receptor and potentially another transcriptional regulator via a cis -regulatory element in the ptr-8 promoter to repress its expression, thus ensuring proteostasis and prolonged longevity (Fig. 6 ). These findings reveal the key role of a lipid metabolic enzyme in nutrients-mediated modulation of ageing and elucidate the underlying transcriptional regulation mechanisms. DR is an effective method to delay ageing in many species. Previous studies have identified key mediators of DR-induced longevity, many of which are transcriptional regulators. However, it has not been clear whether metabolic enzymes play key roles in the response to DR. Lipid metabolism plays important roles in both health and diseases. It has been well-documented that obesity is associated with many pathologies. Intriguingly, many long-lived C. elegans mutants, such as daf-2 , rsks-1 , and glp-1 , show increased lipid accumulation, whereas certain longevity mutant such as eat-2 , has reduced lipid levels [34] . Lipid metabolism is a very complex and dynamic process including synthesis, breakdown, transportation, and so on. In this study, we set out to characterize the roles of lipid metabolic enzymes in DR-induced longevity by a targeted RNAi screen of the acs family of genes, which are involved in the rate-limiting step of fatty acid metabolism [20] . We found that ACS-20 is required for DR-induced lifespan and healthspan extension (Fig. 1 ). Unlike some mediators of DR that are functional only in certain DR regimens, ACS-20 is required for the lifespan extension by bacterial food dilution or the eat-2 genetic mimic of DR, suggesting it is bona fide mediator of DR. The temporospatial analysis reveals that ACS-20 functions in the epidermis during development to regulate DR-induced longevity, which is consistent with the endogenous expression patterns of ACS-20 (Fig. 2 ). It is intriguing that certain interventions, such as perturbation of the mitochondrial electron transport chain and removal of the germline via physical or genetic methods, are required to be performed during development to affect C. elegans ageing [35] , [36] . The acs-20 deletion mutant does not cause developmental arrest or sterility, suggesting it might not cause sickness in general. The epidermal tissue not only serves as a barrier for protection, but also plays important roles in body morphology and physiology, such as secretion, lipid storage, glia-like functions, and innate immunity [37] , [38] . It has been reported that reduced insulin-like signaling functions through the SKN-1 transcription factor to delay ageing via collagen genes, the expression products of which are secreted by epidermal cells to form the cuticle in C. elegans [39] . Here we found acs-20 and the downstream genes all function in the epidermis to regulate the effect of nutrients on longevity, which highlights the importance of this tissue for further exploration in ageing research. Transcriptome profiling reveals that genes upregulated in the eat-2; acs-20 double mutant are enriched with UPR ER -related genes, and the acs-20 mutant is more sensitive to the ER stress-inducing drugs tunicamycin, DTT and thapsigargin (Fig. 3 and Supplementary Fig. 4 ). These results suggest that the acs-20 mutant might have disrupted proteostasis, which has been associated with ageing and age-related degenerative diseases [40] . To further explore the underlying molecular mechanisms, we performed an RNAi-based genetic screen of genes upregulated in the short-lived eat-2; acs-20 double mutant for the lifespan extension phenotype. PTR-8, a C. elegans ortholog of Patched from the Hedgehog pathway, was identified as a key downstream regulator of lifespan and proteostasis (Fig. 4 ). The Hedgehog pathway plays important roles during development. However, this signaling has certain key components missing but significant expansion of Hedgehog receptor genes in C. elegans [41] . Whether this non-canonical function of PTR-8/Patched in healthy ageing is conserved in higher organisms should be explored in future studies. Since ptr-8 is transcriptionally elevated in the eat-2; acs-20 double mutant, we performed a targeted RNAi screen of 757 transcription factor-related genes and identified NHR-23 as a transcriptional repressor of ptr-8 . Consistent with the gene expression results, RNAi knockdown of NHR-23 in the epidermis also blocks DR-induced longevity (Fig. 5 ). NHR-23 is orthologous to the nuclear receptor RORA, which plays an important role in circadian clock regulation. It has been reported that inhibition of key regulators of the circadian clock blocks DR-induced longevity through affecting lipid turnover in Drosophila [42] . Although C. elegans does not have a 24-h rhythm, certain circadian clock genes are conserved, and they are involved in the regulation of developmental timing in the epidermis, such as molting. Our findings highlight the importance of circadian clock genes in DR-induced healthy ageing. To further dissect the transcriptional regulation of ptr-8 by NHR-23, we mapped the cis- regulatory element to a specific region of the ptr-8 promoter. Although NHR-23 directly binds to this region, gene expression studies suggest that NHR-23 might function through another transcriptional regulator to affect ptr-8 expression indirectly (Fig. 5 and Fig. 6 ). It will be interesting to identify this unknown transcriptional regulator and further elucidate the mechanisms of gene expression in future studies. Does ACS-20 play regulatory roles in other long-lived mutants? To address this question, we crossed the acs-20 mutation into the long-lived daf-2 (IGF-1 receptor), glp-1 (Notch receptor), rsks-1 (ribosomal S6 kinase), and isp-1 (iron-sulfur protein of the mitochondrial ETC complex III) mutants, which represent reduced insulin/IGF-1 signaling [43] , [44] , germline deficiency [36] , reduced TOR signaling [45] , and perturbation of the mitochondrial electron transport chain [46] , respectively. Survival assays show that the acs-20 mutation partially blocks the lifespan extension by daf-2 and glp-1 , whereas it completely suppresses the prolonged longevity by rsks-1 or isp-1 (Supplementary Fig. 5 ). These data suggest that the effects of acs-20 on longevity are context-dependent, and the suppression of longevity by acs-20 is unlikely due to sickness in general. The relationship between lipid metabolism and longevity is complicated. Both increased and decreased lipid accumulation were originally associated with prolonged longevity, but more and more evidence indicate that it is not the level of lipids but the active utilization of lipids that contributes to the lifespan extension [34] . Our lipid staining and lipid droplets GFP reporter assays show that the acs-20 mutation does not have a strong effect on neutral lipid levels in the intestine or epidermis (Supplementary Fig. 3 ). Further biochemical analysis shows that inhibition of acs-20 does not change the levels of most fatty acids, but it does affect certain phospholipids and sphingolipids (Supplementary Fig. 3e-g ). It was reported that ACS-3, another long-chain acyl-CoA synthetase, functions in epidermal cells to direct the biosynthesis of phospholipid ligands for the NHR-25 nuclear receptor in C. elegans [47] . It will be interesting to determine whether certain lipid metabolic products of ACS-20 function as the ligand for NHR-23 to regulate ptr-8 expression, proteostasis, and longevity in future studies. Our findings demonstrate that ACS-20, NHR-23, and PTR-8 all function in the epidermis to regulate proteostasis and longevity under DR conditions. Since the polyQ model used to assess proteostasis is expressed in muscle cells and the lifespan phenotypes occur at the whole animal level, it is plausible that these regulators might work through cell-non-autonomous manner to affect ageing. It will be interesting to further analyze the molecular events downstream of PTR-8 via genetic and genomic approaches to better understand how non-canonical Hedgehog signaling affects ageing in response to nutrients. In summary, we have identified a fatty acid metabolic enzyme as the key modulator of healthy ageing in response to nutrients. The underlying mechanisms involve transcriptional regulation of the Hedgehog signaling and maintenance of proteostasis. Further characterization of the molecular details should help to better understand the mechanisms of ageing and develop pharmaceutical interventions to delay ageing. C. elegans strains All strains were maintained on NGM agar plates seeded with E. coli OP50 at 20 °C. A list of C. elegans strains used in this study can be found in Supplementary Data S 2 . Lifespan assay Lifespan assays were performed at 20 °C unless otherwise stated. To prevent progeny production, 20 μg/ml (+)-5-fluorodeoxyuridine (FUdR) was added onto NGM plates during the reproductive period (Day 1–7 of adulthood). The first day of adulthood is day 1 on survival curves. Animals were scored as alive, dead, or lost every other day. Animals that did not respond to gentle touch were scored as dead. Animals that died from causes other than ageing, such as sticking to the plate walls, internal hatching or bursting in the vulval region, were scored as lost. Lifespan assays under differential nutrient conditions were performed using the modified solid DR method [14] . Day 1 adult animals were treated with bacterial food at different concentrations and survival was monitored at 25 °C. Kaplan–Meier survival curves were plotted for each lifespan assay, and statistical analyses (log-rank tests). RNAi by feeding RNAi experiments were performed by feeding worms E. coli strain HT115 (DE3) transformed with either the empty vector L4440 as the control or gene-targeting constructs from the C. elegans Ahringer RNAi Collection [48] . Overnight bacterial culture in LB supplemented with Ampicillin (100 μg/ml) at 37 °C was seeded onto NGM plates containing IPTG (1 mM) and Ampicillin (100 μg/ml) and incubated at the room temperature overnight to induce double-stranded RNAs production. Embryos or L1 larvae were placed on RNAi plates and incubated at 20 °C until L4 or adulthood to score phenotypes. For nhr-23 , the RNAi treatment was initiated at the L2 stage to avoid sickness produced by nhr-23 knockdown. Stress resistance assays For the heat stress assays, synchronized day 1 adult worms were incubated at 35 °C for 10 h before counting the numbers of alive or dead animals. For the ER stressor tolerance assays, gravid adults were put on the plates supplemented with different concentrations of tunicamycin (0, 0.25, 0.50 μg/ml), DTT (0, 25, 50 μg/ml) or thapsigargin (0, 25, 50 μg/ml) to lay eggs for 1 h. The developmental stages of the progeny were quantified when most animals from the control group have reached to the L4 stage or beyond. Fluorescence imaging of C. elegans Animals were anesthetized in 1% sodium azide and immediately imaged. For the ptr-8 transcriptional reporters, animals were imaged with a Leica MC165 FC dissecting microscope equipped with a Leica DFC450 C digital camera. For ACS-20::GFP or Q35::YFP, animals were imaged with a Zeiss LSM880 confocal microscope equipped with a 40X/1.3 W objective controlled by the ZEN software (Carl Zeiss). For GFP or YFP, a 488 nm laser was used for excitation, and signals were collected with a 500-550 nm emission filter. In all the imaging studies, images within the same figure panel were taken with the same exposure time and adjusted with identical parameters using Adobe Photoshop or ImageJ. Western blot and antibodies Roughly equal numbers of synchronized L4 animals were manually transferred into the lysis buffer (150 mM NaCl, 1 mM EDTA, 0.25% SDS, 1.0% NP-40, 50 mM Tris-HCl [pH7.4], Roche complete protease inhibitors and phosSTOP phosphatase inhibitors) supplemented with the 4 × SDS loading buffer and immediately frozen at -80 °C. Samples were boiled for 10 min before resolving on precast SDS-PAGE gels (GenScript). Bands of interests were quantified using the ImageJ software and normalized to the intensities of α-tubulin, the internal control. Antibodies used in Western blots include monoclonal anti-FLAG (Sigma, 1804) and monoclonal anti-Tubulin Alpha (Sigma, T6074), which are both used at 1:10,000 dilution. Filter trap assays Synchronized Day 3 adult worms were collected with the M9 buffer, and immediately frozen with liquid nitrogen. Worm pellets were thawed on ice, and worm extracts were generated by sonication in the FTA buffer [50 mM Hepes (pH 7.4), 1 mM EDTA, 150 mM NaCl, and 1% Triton X-100] supplemented with the EDTA-free protease inhibitor cocktail (Roche). Worm debris was removed by centrifugation at 8000 g for 15 min at 4 °C. 100 μg of protein extracts were supplemented with SDS at the final concentration of 0.5% and loaded onto a cellulose acetate membrane with 0.22 μm pore size assembled in a slot blot apparatus (Bio-Rad). The membrane was then washed with 0.2% SDS and SDS-resistant protein aggregates were assessed by immunoblotting using antibodies against GFP (AMSBIO, TP401, 1:500 dilution). Extracts were also analyzed by SDS-PAGE and Western blots with the anti-GFP (AMSBIO, TP401, 1:500 dilution) and anti-Tubulin Alpha (Sigma, T6074, 1:10,000 dilution) primary antibodies, as well as the goat anti-mouse IgG (H + L) HRP secondary antibodies (Bioworld BS12478, dilution 1:10,000). The intensities of bands from filter trap and Western blot were measured with ImageJ. mRNA-Seq and bioinformatics analysis Three biological replicates of total mRNAs from N2, eat-2 , acs-20 , and eat-2; acs-20 mutant L4 larvae were sent to Berry Genomics for library construction and pair-ended sequencing with the length of 100 nucleotides, 11.5 million reads per sample on a HiSeq2000 machine (Illumina). Reads were aligned to the C. elegans genome (WS220) using the spliced-junction mapper TopHat2 [49] . Aligned reads were counted per gene using the python script HTseq [50] . Differentially expressed genes were determined via DESeq2. The mRNA-Seq data have been deposited at the NCBI under accession number GSE125718. GO analysis GO analyses was performed using Metascape ( https://metascape.org/ ). Terms with a p < 0.01, a minimum count of 3, and an enrichment factor >1.5 were collected and grouped into clusters based on their membership similarities [51] . RT-qPCR Synchronized L4 animals were collected for total RNA extractions using the Trizol reagent (Takara) and Direct-zol RNA mini prep kit (ZYMO Research). The cDNA was synthesized by the reverse transcription system (Takara). The SYBR Green dye (Takara) was used for qPCR reactions carried out in triplicates on a Roche LightCycler 480. Relative gene expression levels were calculated using the 2 -ΔΔCt method [52] . RT-qPCR experiments were performed at least three times with consistent results using independent RNA preparations. CRISPR/Cas9 alleles generation CRISPR engineering with a self-excising drug selection cassette (SEC) were performed to knock-in GFP::3 × FLAG at the C-terminal of ACS-20 and NHR-23 using the homologous recombination approach [53] . The injection mix contained two plasmids that drive expression of two different Cas9-sgRNAs (50 ng/ml), a selection marker pCFJ90 (P myo-2::mCherry::unc-54 -3’-UTR) (2.5 ng/ml, Addgene #19327) and a homologous recombination plasmid (50 ng/ml). 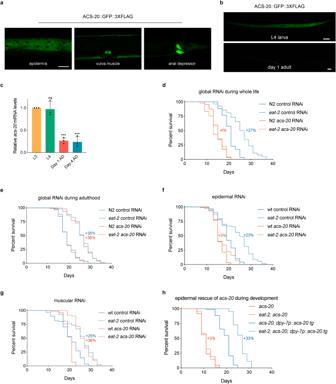Fig. 2: ACS-20 functions in the epidermis during development to regulate DR-induced lifespan extension. aRepresentative photographs of the endogenous ACS-20::GFP::3✕FLAG expression in different tissues. Scale bar, 20 μm.bRepresentative photographs of ACS-20::GFP expression in the fourth larval stage (L4) and day 1 adulthood. Scale bar, 50 μm.cRT-qPCR quantification ofacs-20mRNAs at different stages. Data are represented as mean ± SD (n= 3). ns,p= 0.9880; ***p< 0.001 (One-way ANOVA with Turkey’s multiple comparisons test).d,eSurvival curves of N2 andeat-2mutant animals treated with the global control oracs-20RNAi in whole life (d) or adulthood (e). N2 vs.eat-2with the control RNAi treatment,p< 0.0001 (whole life, adulthood); N2 vs.eat-2with theacs-20RNAi treatment,p= 0.3093 (whole life),p< 0.0001 (adulthood) (log-rank tests).f,gSurvival curves of wild type (wt) andeat-2mutant animals treated with the epidermal (f) or muscular (g) control oracs-20RNAi. wt vs.eat-2with the control RNAi treatment,p< 0.0001 (epidermal RNAi, muscular RNAi); wt vs.eat-2with theacs-20RNAi treatment,p= 0.0662 (epidermal RNAi),p< 0.0001 (muscular RNAi) (log-rank tests).hSurvival curves ofacs-20andeat-2; acs-20mutants with or without theacs-20transgene driven by the epidermis-specificdpy-7promoter.acs-20vs.eat-2; acs-20,p= 0.9773 (without the transgene),p< 0.0001 (with the transgene) (log-rank tests). Percentages indicate changes in mean lifespan induced by theeat-2mutation. Source data are provided as a Source Data file. To generate the sgRNA plasmids, primers were designed with the CRISPR DESIGN tool ( https://zlab.bio/guide-design-resources ) and inserted into the pDD162 vector (Addgene #47549) using the site-directed mutagenesis kit (TOYOBO SMK-101). The ccdB sequences from the pDD282 vector (Addgene #66823) were replaced with two homologous arms (500–700 bp) to generate the repair template FP-SEC plasmid. Injected animals and their progeny were treated with Hygromycin B (350 mg/ml) to select successful knock-in events. Hygromycin B resistant roller animals were tested by PCR genotyping. The SEC was removed by heat shock and homozygous knock-in alleles were confirmed by PCR and DNA sequencing. ChIP-qPCR Synchronized L4 larvae were washed with the M9 buffer for three times and fixed with 37% formaldehyde for 30 min followed by stopping with 2.5 M Glycine for 15 min. Samples were washed twice with 1 X PBS, once with the CL-WS1 buffer [50 mM HEPES/KOH pH 7.5, 150 mM NaCl, 0.1% sodium deoxycholate, 1% Triton X-100, 1 mM EDTA, 1 mM PMSF, EDTA-free protease inhibitor cocktail], ground in liquid nitrogen, resuspended in 2 ml ice-cold CL-Lysis buffer [50 mM HEPES-KOH pH 7.5, 150 mM NaCl, 0.1% sodium deoxycholate, 1% Triton X-100, 0.1% SDS, 1 mM EDTA, 1 mM DTT, 1 mM PMSF, EDTA-free protease inhibitor cocktail], and sonicated using a Bioruptor UCD-200 at high mode for 15 cycles of 30 s on and 30 s off. Samples were then centrifuged at 18,000 g for 15 min at 4 °C, and the supernatant was transferred to a new tube. 5% of the extracts were saved as input sample, and 5 μg of chromatin as ChIP samples were incubated with GFP-Trap Dyna beads (ChromoTek, # gtd) for 1 h, and then washed twice with the CL-WS2 buffer [50 mM HEPES/KOH pH 7.5, 1 M NaCl, 0.1% sodium deoxycholate, 1% Triton X-100, 1 mM EDTA, 1 mM PMSF, EDTA-free protease inhibitor cocktail], once with the CL-WS3 buffer [10 mM Tris·HCl pH 8.0, 0.25 M LiCl, 1% sodium deoxycholate, 1% NP-40, 1 mM EDTA, 1 mM PMSF, EDTA-free protease inhibitor cocktail], once with the CL-WS4 buffer [10 mM Tris·HCl, pH 8.0, 1 mM EDTA]. 100 μl of the CL-Elution buffer [10 mM Tris·HCl, pH 8.0, 250 mM NaCl, 1% SDS, 1 mM EDTA] was added to the sample and incubated for 30 min at 65 °C. ChIP samples were vortexed, and the supernatants were collected. 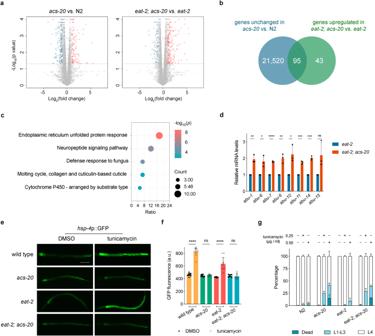Fig. 3: Theacs-20mutation causes ER stress under DR. aVolcano plots of differentially expressed genes in theacs-20vs. N2 andeat-2; acs-20vs.eat-2data sets. Red and blue points represent genes with significantly increased or decreased expression, respectively (p< 0.01, Wald tests with Bonferroni corrections).bA Venn diagram comparing genes upregulated ineat-2; acs-20vs.eat-2and genes not differentially expressed inacs-20vs. N2.cSignificantly enriched Gene Ontology (GO) terms (hypergeometric tests with Benjamini-Hochberg corrections) for genes significantly upregulated in theeat-2; acs-20mutant compared to theeat-2mutant.dRT-qPCR quantification ofabugenes ineat-2andeat-2; acs-20mutant animals. Data are represented as mean ± SD (n= 3). ****p< 0.0001; ***p< 0.001; **p< 0.01; *p< 0.05; ns,p= 0.0598 (two-tailedt-tests).e,fRepresentative photographs of the ER stress reporterhsp-4p::gfpexpression in wild-type,acs-20,eat-2, andeat-2; acs-20animals treated with DMSO or tunicamycin (e) and quantification of the GFP fluorescence intensities (a.u. arbitrary unites). Data are represented as mean ± SD (n= 10). ****p< 0.0001; ns,acs-20 p> 0.9999,eat-2; acs-20 p= 0.9993 (One-way ANOVA with Turkey’s multiple comparisons test). Scale bar, 200 μm.gPercentages of N2,acs-20,eat-2, andeat-2; acs-20mutant animals that died (dead), developmentally arrested (L1-L3) or completed development (L4) upon 0, 0.25 or 0.50 μg/ml tunicamycin treatments. Data are represented as mean ± SD (n= 3). For animals that completed development upon tunicamycin treatment, N2 vs.acs-20,p< 0.01;eat-2vs.eat-2; acs-20,p< 0.0001 (Two-way ANOVA with Turkey’s multiple comparisons test). Source data are provided as a Source Data file. RNaseA was then added to both the ChIP and input samples, and incubated for 1 h at 37 °C. The crosslink was reversed with proteinase K at 65 °C for >4 h. DNA was purified with the Qiagen Maxtract kit (Qiagen, #129046) and used as templates for qPCR. Oligo sequences A list of oligo sequences used for qPCR and CRISPR/Cas9 experiments in this study can be found in Supplementary Data S 3 . 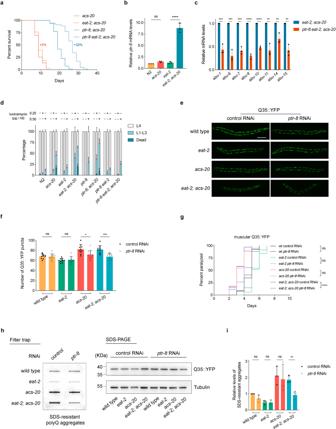Fig. 4: Elevated PTR-8 expression inacs-20disrupts the protective effect of DR on lifespan and proteostasis. aSurvival curves ofacs-20,eat-2; acs-20,ptr-8; acs-20, andptr-8 eat-2; acs-20.acs-20vs.eat-2; acs-20,p= 0.0995;ptr-8; acs-20vs.ptr-8 eat-2; acs-20,p< 0.0001 (log-rank tests). Percentages indicate changes in mean lifespan induced byeat-2.bRT-qPCR quantification ofptr-8mRNAs in N2,acs-20,eat-2, andeat-2;acs-20. Data are represented as mean ± SD (n= 3). ****p< 0.0001; ns,p= 0.7886 (One-way ANOVA with Turkey’s multiple comparisons test).cRT-qPCR quantification ofabugenes ineat-2; acs-20andptr-8 eat-2; acs-20. Data are represented as mean ± SD (n= 3). ****p< 0.0001; ***p< 0.001; **p< 0.01 (two-tailedt-tests).dPercentages of N2,acs-20,eat-2,eat-2; acs-20,ptr-8,ptr-8; acs-20,ptr-8 eat-2, andptr-8 eat-2; acs-20that died (dead), developmentally arrested (L1-L3) or completed development (L4) upon 0, 0.25 or 0.50 μg/ml tunicamycin treatment. Data are represented as mean ± SD (n= 3). For animals that completed development upon tunicamycin treatment,eat-2vs.eat-2; acs-20,p< 0.0001;eat-2; acs-20vs.ptr-8 eat-2; acs-20,p< 0.0001 (Two-way ANOVA with Turkey’s multiple comparisons test).e,fRepresentative photographs of wild-type,acs-20,eat-2, andeat-2; acs-20animals expressing muscular Q35::YFP treated with the control orptr-8RNAi (e) and quantification of the Q35::YFP punctae (f). Data are represented as mean ± SD (n= 10). ****p< 0.0001; **p< 0.01 (One-way ANOVA with Turkey’s multiple comparisons test). Scale bar, 100 μm.gParalysis analysis of the wild-type,eat-2,acs-20, andeat-2; acs-20mutant animals expressing muscular Q35::YFP with control orptr-8RNAi. ****p< 0.0001; ns,p> 0.05 (log-rank tests).h,iImmuno-blots (h) and quantification (i) of the SDS-resistant Q35::YFP aggregates, total Q35::YFP, and tubulin in the wild-type,eat-2,acs-20, andeat-2; acs-20with control orptr-8RNAi. Data are represented as mean ± SD (n= 3). **p< 0.01; ns,p> 0.05 (One-way ANOVA with Turkey’s multiple comparison tests). Source data are provided as a Source Data file. Statistical analysis All statistical analyses were preformed using two-tailed t -tests, one-way or two-way ANOVA with Turkey’s multiple comparisons test, and log-rank tests as reported in figure legends and Source Data. Bar graphs are presented as mean ± SD with p < 0.05 considered as significant differences. 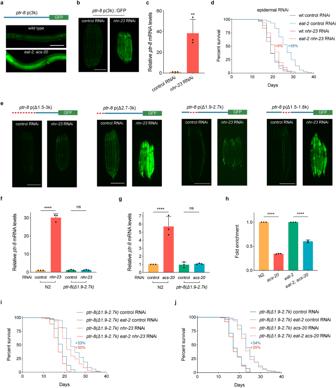Fig. 5: NHR-23/RORA mediates the effect ofacs-20onptr-8expression and lifespan. aRepresentative photographs of theptr-8p(3k)::GFP reporter expression in wild-type andeat-2; acs-20animals. Scale bar, 50 μm.bRepresentative photographs of theptr-8p(3k)::GFP expression in animals treated with the control ornhr-23RNAi. Scale bar, 200 μm.cRT-qPCR quantification ofptr-8mRNA levels in wild-type animals treated with the control ornhr-23RNAi. Data are represented as mean ± SD (n= 3). **p= 0.0084 (two-tailedt-test).dSurvival curves of wild type (wt) andeat-2mutant animals treated with the epidermis-specific control ornhr-23RNAi. wt vs.eat-2: control RNAi,p< 0.0001;nhr-23RNAi,p< 0.01 (log-rank tests).eRepresentative photographs of theptr-8p(Δ1.5-3 k)::GFP,ptr-8p(Δ2.7-3 k)::GFP,ptr-8p(Δ1.9-2.7 k)::GFP, andptr-8p(Δ1.5-1.8 k)::GFP expression in animals treated with the control ornhr-23RNAi. Scale bar, 200 μm.f,gRT-qPCR quantification ofptr-8mRNA levels in N2 and theptr-8p(Δ1.9-2.7 k) mutant animals treated with either control vs.nhr-23RNAi (g) or control vs.acs-20RNAi (h). Data are represented as mean ± SD (n= 3). ****p< 0.0001; ns,p= 0.9972 (nhr-23RNAi),p= 0.9972 (acs-20RNAi) (One-way ANOVA with Turkey’s multiple comparisons test).hChIP-qPCR quantification of the relative enrichment of NHR-23::GFP binding with theptr-8promoter region (1861–1958 bp) in N2,acs-20,eat-2andeat-2; acs-20. The fold enrichment was normalized by the input DNA. Data are represented as mean ± SD (n= 3). ****,p< 0.0001 (two-tailedt-tests).i,jSurvival curves ofptr-8p(Δ1.9-2.7 k) andptr-8p(Δ1.9-2.7 k)eat-2mutant animals treated with the control vs.nhr-23RNAi (i) oracs-20RNAi (j).ptr-8p(Δ1.9–2.7 k) vs.ptr-8p(Δ1.9–2.7 k)eat-2: control RNAi,p< 0.0001;nhr-23RNAi,p< 0.0001;acs-20RNAi,p< 0.0001 (log-rank tests). Percentages indicate changes in mean lifespan induced by theeat-2mutant. Source data are provided as a Source Data file. 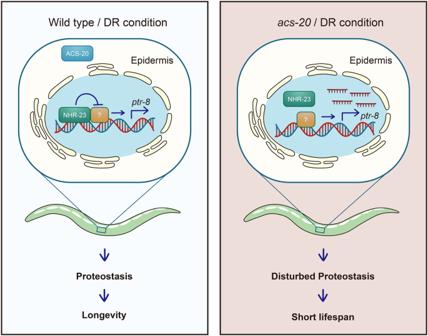Fig. 6: Schematic representation on the regulation of DR-induced healthy ageing by ACS-20, NHR-23, and PTR-8. ACS-20 functions in the epidermis during development to regulate DR-induced lifespan extension. In the presence of ACS-20, the NHR-23/RORA nuclear hormone receptor functions with an unknown factor to restrict the expression of PTR-8/Patched via acis-regulatory element to maintain proteostasis and promote healthy ageing under DR. In the absence of ACS-20, NHR-23-mediated transcriptional repression ofptr-8is abolished. Overexpression of PTR-8 results in disrupted proteostasis and elevated ER stress, which block the lifespan extension produced by DR. Reporting summary Further information on research design is available in the Nature Portfolio Reporting Summary linked to this article.